Electrochemically tunable thermal conductivity of lithium cobalt oxide Using time-domain thermoreflectance, the thermal conductivity and elastic properties of a sputter deposited LiCoO 2 film, a common lithium-ion cathode material, are measured as a function of the degree of lithiation. Here we report that via in situ measurements during cycling, the thermal conductivity of a LiCoO 2 cathode reversibly decreases from ~5.4 to 3.7 W m −1 K −1 , and its elastic modulus decreases from 325 to 225 GPa, as it is delithiated from Li 1.0 CoO 2 to Li 0.6 CoO 2 . The dependence of the thermal conductivity on lithiation appears correlated with the lithiation-dependent phase behaviour. The oxidation-state-dependent thermal conductivity of electrolytically active transition metal oxides provides opportunities for dynamic control of thermal conductivity and is important to understand for thermal management in electrochemical energy storage devices. Controlling the flow of heat through materials is important for many technologies [1] , [2] . Although materials with high and low thermal conductivities are available, materials with variable and reversible thermal conductivities are rare, and other than high pressure experiments, only small reversible modulations in thermal conductivities have been reported [3] , [4] , [5] . Various forms of nanostructuring [6] , [7] , [8] , [9] , [10] , [11] , [12] , [13] , including forming multilayer structures with high interface densities [14] , [15] , [16] , have been shown to be effective strategies for reducing the thermal conductivity of non-metals. However, because these nanostructures are static, this has not been a route to dynamic modulation of thermal properties. Here we show, via in situ measurements, electrochemical modulation of the thermal conductivity of a sputtered film of Li x CoO 2 over the unprecedented range of 5.4 to 3.7 W m −1 K −1 for x =1.0 to 0.6. Via ex situ measurements on a sample annealed at a higher temperature than possible for the in situ samples, the thermal conductivity ratio between the lithiated and delithiated state is observed to exceed 2.7. Experimental system Li x CoO 2 is selected because of its reversible lithiation characteristics, and because it is widely used as a cathode material in high-energy density Li-ion batteries. In our experiments, the Li content is controlled by charging and discharging using galvanostatic cycling with the potential limit technique [17] over a potential range of 3.0–4.2 V. Metallic Li is used as the counter and quasi-reference electrode. Thermal conductivity is measured using time-domain thermoreflectance (TDTR) [1] , [18] . As illustrated in Fig. 1a , the experimental system comprises a transparent substrate consisting of plasma-enhanced chemical vapour deposition (PECVD) deposited SiO 2 on sapphire, coated with an Al layer that acts as the electrochemical current collector, thermal transducer and thermometer. LiCoO 2 is sputter deposited on this stack. Sapphire is selected for the substrate because of its optical transparency and high thermal conductivity, which limits the steady-state temperature rise to 3 K during the TDTR measurement (see Supplementary Information ),which is small enough to avoid significant changes to the Li x CoO 2 electrochemical properties. The SiO 2 layer suppresses the transient diffusion of heat from the Al layer to the sapphire substrate and ensures that about 75% (see Supplementary Information ) of the heat generated by pump laser beam initially dissipates into the Li x CoO 2 , enabling accurate measurement of the thermal conductivity of the Li x CoO 2 . Between pulses, this heat dissipates into the sapphire substrate, minimizing the steady-state temperature increase. 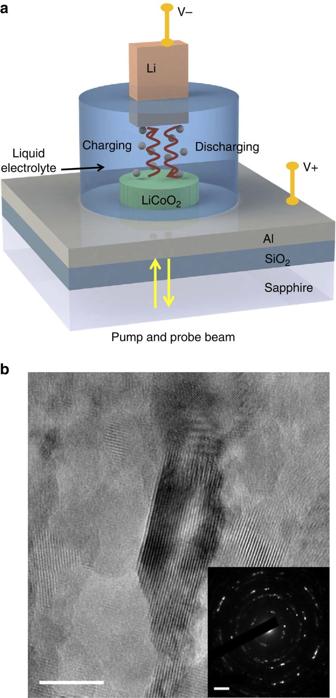Figure 1: Experimental system. (a) Schematic of thein situmeasurement cell consisting of ~500 nm of LiCoO2, 70 nm of Al (the transducer) and 100 nm of SiO2(thermal isolation layer) on a sapphire substrate. The LiCoO2is immersed in a liquid electrolyte of 1:1 ethylene carbonate and dimethyl carbonate containing 1 M LiClO4. The LiCoO2thin film was sputter deposited through a metal hard mask to define its area. (b) Cross-sectional HRTEM image of the LiCoO2film after 500 °C annealing in air. The polycrystalline nature and random texturing can be seen from both the lattice fringes and the selected area diffraction (inset). The scale bar inbis 10 nm and the scale bar in the inset ofbis 2 nm−1. Figure 1: Experimental system. ( a ) Schematic of the in situ measurement cell consisting of ~500 nm of LiCoO 2 , 70 nm of Al (the transducer) and 100 nm of SiO 2 (thermal isolation layer) on a sapphire substrate. The LiCoO 2 is immersed in a liquid electrolyte of 1:1 ethylene carbonate and dimethyl carbonate containing 1 M LiClO 4 . The LiCoO 2 thin film was sputter deposited through a metal hard mask to define its area. ( b ) Cross-sectional HRTEM image of the LiCoO 2 film after 500 °C annealing in air. The polycrystalline nature and random texturing can be seen from both the lattice fringes and the selected area diffraction (inset). The scale bar in b is 10 nm and the scale bar in the inset of b is 2 nm −1 . Full size image The thermal transport properties of the Li x CoO 2 film are analysed by solution of bidirectional heat diffusion equation in cylindrical coordinates for a multi-layered geometry [19] . Thermal conductivity, specific heat and thickness of each layer are parameters for bidirectional thermal modelling. We determine the thermal conductivity of the Li x CoO 2 layer by the best fit between the calculation of the thermal model and the measured TDTR data (see Supplementary Information ). Achieving high-quality LiCoO 2 in contact with the Al transducer is a challenge because of the low-melting point of Al and its susceptibility to oxidation. LiCoO 2 films sputter deposited at room temperature are largely amorphous and exhibit poor Li intercalation capacities. Li ion intercalation reaches maximum capacity and full reversibility only when LiCoO 2 is crystallized at or above 700 °C in an oxygen atmosphere [20] . However, these conditions are incompatible with the Al electrode favourable for the in situ TDTR measurements. Pt, which has been used for TDTR studies [21] , was considered instead of Al; however, Pt did not provide a sufficient optical response [22] , [23] , and thus was not used. As a compromise, we chose an annealing temperature of 500 °C that affords good LiCoO 2 crystallinity and electrochemical properties, while avoiding aluminum oxidation. After annealing at 500 °C, the LiCoO 2 films are polycrystalline ( Fig. 1b ), have a discharging capacity of ~95 mA h g −1 (calculated from the data in Fig. 2a ), compared with 117 mA h g −1 for films annealed at 700 °C ( Supplementary Fig. 1 ) and exhibit a clear Li ion intercalation reaction at ~3.9 V ( Supplementary Fig. 3 ). Although transmission electron microscopy (TEM) studies ( Fig. 1b ) do not indicate texturing, X-ray diffraction ( Supplementary Fig. 8 ) indicates the 500 °C annealed LiCoO 2 film shows preferred (101) and (104) texture. The effect of texturing on thermal conductivity is discussed in the Supplementary Information . 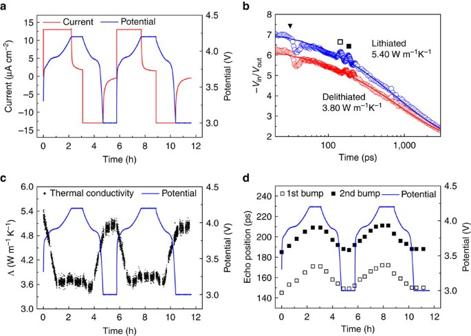Figure 2: Electrochemical, thermal and acoustic properties of the LixCoO2film. (a) Electrochemical cycling data during TDTR measurements. The LixCoO2was galvanostatically cycled between 3.0 and 4.2 V at 13 μA cm−2(~6 h per cycle). At the end of each charge and discharge step the potential is held constant for 1 h to allow the system to approach equilibrium (the current after 1 h is less than 10% of the galvanostatic charging and discharging current). The galvanostatic C-rate is about 0.3C, and the specific capacities of the electrode are 129 and 95 mA h g−1for charge and discharge of first cycle shown and 115 and 93 mA h g−1for second cycle, respectively. The LiCoO2is pre-cycled three times before TDTR measurements. (b) TDTR data (open circles) and thermal conductivity fit (lines) for representative lithiated (x=1.0) and delithiated (x=0.6) LixCoO2. The ratio of the in-phase and out-of-phase signals from the rf lock-in amplifier, −Vin/Vout, represents the thermal decay as a function of time after the pump beam heats the Al layer. (c) Thermal conductivity and potential profiles as a function of time under the cycling profile shown ina. The voltage ratio, −Vin/Vout, at 30 ps (indicated as a black inverse triangle inb) provides the real-time thermal conductivity during cycling. (d) The acoustic echo positions as a function of reaction time (indicated by the open and filled squares inb) under the cycling profile shown ina. Figure 2: Electrochemical, thermal and acoustic properties of the Li x CoO 2 film. ( a ) Electrochemical cycling data during TDTR measurements. The Li x CoO 2 was galvanostatically cycled between 3.0 and 4.2 V at 13 μA cm −2 (~6 h per cycle). At the end of each charge and discharge step the potential is held constant for 1 h to allow the system to approach equilibrium (the current after 1 h is less than 10% of the galvanostatic charging and discharging current). The galvanostatic C-rate is about 0.3C, and the specific capacities of the electrode are 129 and 95 mA h g −1 for charge and discharge of first cycle shown and 115 and 93 mA h g −1 for second cycle, respectively. The LiCoO 2 is pre-cycled three times before TDTR measurements. ( b ) TDTR data (open circles) and thermal conductivity fit (lines) for representative lithiated ( x =1.0) and delithiated ( x =0.6) Li x CoO 2 . The ratio of the in-phase and out-of-phase signals from the rf lock-in amplifier, − V in / V out , represents the thermal decay as a function of time after the pump beam heats the Al layer. ( c ) Thermal conductivity and potential profiles as a function of time under the cycling profile shown in a . The voltage ratio, − V in / V out , at 30 ps (indicated as a black inverse triangle in b ) provides the real-time thermal conductivity during cycling. ( d ) The acoustic echo positions as a function of reaction time (indicated by the open and filled squares in b ) under the cycling profile shown in a . Full size image Measured Li x CoO 2 thermal properties Figure 2b presents representative in situ TDTR data comparing thermal conductivity of lithiated and delithiated Li x CoO 2 films. The thermal conductivity of Li 1.0 CoO 2 is 5.4 W m −1 K −1 , which reduces to 3.7 W m −1 K −1 when the film is delithiated to Li 0.6 CoO 2 . Complete TDTR data sets from −20 ps to 3,600 ps take a few minutes to collect. To obtain nearly continuous thermal conductivity measurements during galvanostatic delithiation and lithiation, the delay time is fixed at 30 ps, and the in-phase and out-of-phase signal from the lock-in amplifier is recorded and converted every 6 s to thermal conductivity [24] (see Supplementary Information for details of experimental measurements). Figure 2c gives the thermal conductivity of Li x CoO 2 during delithiation (0–3 h and 6–9 h) and lithiation (3–6 h and 9–12 h) over the range of x =1.0 to x =0.6. The thermal conductivity decreases from ~5.4 to 3.7 W m −1 K −1 during delithiation from x =1.0 to 0.8 and then remains essentially constant with delithiation down to x =0.6 ( Fig. 3a ). During lithiation, the thermal conductivity is reversible. 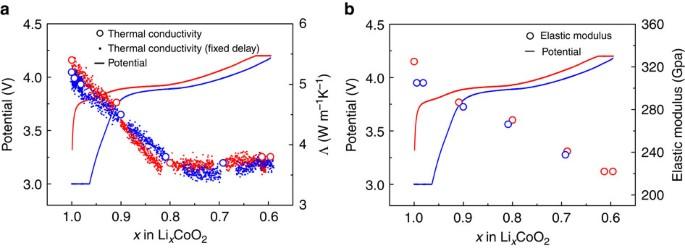Figure 3: Thermal conductivity and longitudinal elastic modulus as a function of LixCoO2lithiation. (a) Thermal conductivity and potential versus Li of LixCoO2as a function ofx. The thermal conductivity is measured using both the full fit to the TDTR data (open circles) and the data at a fixed delay time of 30 ps (solid data points). (b) The lithiation-dependent longitudinal elastic modulus of LixCoO2calculated from the longitudinal speed of sound assuming a LiCoO2density of 5.06 g cm−3(the decrease in density of ~4% going from Li1.0CoO2to Li0.6CoO2was not included in the calculation). In bothaandb, the red data are during delithiation, and the blue during lithiation. Figure 3: Thermal conductivity and longitudinal elastic modulus as a function of Li x CoO 2 lithiation. ( a ) Thermal conductivity and potential versus Li of Li x CoO 2 as a function of x . The thermal conductivity is measured using both the full fit to the TDTR data (open circles) and the data at a fixed delay time of 30 ps (solid data points). ( b ) The lithiation-dependent longitudinal elastic modulus of Li x CoO 2 calculated from the longitudinal speed of sound assuming a LiCoO 2 density of 5.06 g cm −3 (the decrease in density of ~4% going from Li 1.0 CoO 2 to Li 0.6 CoO 2 was not included in the calculation). In both a and b , the red data are during delithiation, and the blue during lithiation. Full size image Ex situ measurements allow for annealing temperatures greater than 500 °C as the Al layer is deposited after Li x CoO 2 annealing, but ex situ measurements do not allow for continuous measurements of thermal conductivity during cycling. The ex situ measured thermal conductivities of Li 0.5 CoO 2 and Li 1.0 CoO 2 films annealed to 700 °C are 3.6 and 9.8 W m −1 K −1 , respectively ( Supplementary Fig. 13 ). Ex situ experiments on the 500 °C annealed Li 1.0 CoO 2 indicate a thermal conductivity of 7.3 W m −1 K −1 (see Supplementary Information ). A hypothesis for the discrepancy between the in situ and ex situ data is included in the Discussion section and the Supplementary Information . Elastic modulus of Li x CoO 2 thin film Along with determination of thermal conductivity, TDTR also enables monitoring of the thickness or elastic properties of a thin layer [25] . The two acoustic echo signals (bumps) visible in Fig. 2b are the result of an acoustic impulse generated by the laser heating and thus thermal expansion of the Al film. The acoustic impulse makes a round trip through the Li x CoO 2 and creates an echo signal when the impulse returns to the substrate. This echo time is presented as a function of x in Fig. 2d . As Li x CoO 2 is delithiated, the two echoes reversibly shift from 145 and 185 ps to 170 and 210 ps. The first echo is an acoustic round trip through the Al and Li x CoO 2 layers and the second echo also includes the acoustic travel time through the SiO 2 layer. In Fig. 2b , at ~40 ps, there is dip indicating an acoustic round trip in the SiO 2 layer. As expected, this dip does not move with lithiation and the time interval between first and second echo is the same as the round trip time of the SiO 2 layer. We can easily rule out changes in electrical conductivities with lithiation, as the mechanism for the changes in thermal conductivity. The room temperature electrical conductivity of Li 1.0 CoO 2 is ~10 −3 S cm −1 and of Li 0.6 CoO 2 is ~10 S cm −1 (refs 26 , 27 , 28 , 29 , 30 ). The Wiedemann–Franz law predicts that as the electrical conductivity increases from ~10 −3 to 10 S cm −1 , the thermal conductivity will increase by 7.3 × 10 −3 W m −1 K −1 . This increase is a factor of ~300 smaller than the observed decrease in thermal conductivity with delithiation of ~1.7 W m −1 K −1 , and has the wrong sign. The thermal conductivity decreases continuously with decreasing lithium content until x =0.8, and then plateaus ( Fig. 3a ). For highly crystalized Li x CoO 2 , it has been reported that a two-phase region exists for 0.75< x <0.93, which corresponds to a voltage plateau during electrochemical cycling [31] . A plausible mechanism for our result is that the two phases (the nearly fully lithiated phase and the partially delithiated phase) have different thermal conductivities, and Li x CoO 2 presents both phases for 1< x <0.8, with an increasing fraction of the lower thermal conductivity phase with decreasing x . Below x =0.8, presumably little of the high thermal conductivity phase is present and the thermal conductivity plateaus. The thermal conductivity data are not a perfect match with the reported phase behaviour: our sample was crystallized at the relatively low temperature of 500 °C, and thus may not exhibit the same phase behaviour as reported inref. [31] . Other possible mechanisms for the changes in thermal conductivity include phonon scattering by the mass disorder created by Li vacancies and phonon scattering by increasing disorder in bond strengths as Li is removed. Both these effects would lead to a lowering of thermal conductivity, and would tend to saturation as the thermal conductivity approaches the minimum thermal conductivity displayed by many strongly disordered materials [32] . That the ex situ measurements reveal a different thermal conductivity for the Li 1.0 CoO 2 for both the 500 and 700 °C annealed samples is not surprising. The ex situ measurements are performed by depositing an Al layer on top of the sputtered LiCoO 2 , and thus are measuring the thermal conductivity of the top of the Li x CoO 2 film as compared with the in situ experiments, which probe the bottom of the film. (The depth sensitivity of a TDTR measurement is approximately given by the penetration depth of the thermal waves generated at the modulation frequency of the pump beam; for these samples, the thermal penetration depth is ~200 nm.) The thermal conductivities of the top and bottom of the sputtered films may be different. It seems reasonable that the higher annealing temperature increases the thermal conductivity, as the grain size of the sample increases with high annealing temperature (see Supplementary Information for TEM images), which may reduce phonon scattering. The relatively low ex situ measured thermal conductivity of the delithiated sample is at first surprising, but again, direct comparison of the quantitative values obtained via in situ and ex situ experiments may not be appropriate because of the changes in texture and grain size. In all cases, the thermal conductivity decreases significantly with delithiation. The change in position of the acoustic echoes with lithium content indicates the Li x CoO 2 film thickness and/or speed of sound varies with lithium content. The unit cell volume increases by only 1.3% going from Li 1.0 CoO 2 to Li 0.6 CoO 2 (ref. 31 ), thus a thickness variation between the lithiated and delithiated states is not sufficient to explain the change in position of the echoes. Assuming a constant Li x CoO 2 thickness of 497 nm, the longitudinal speed of sound changes from 8.01 nm ps −1 for Li 1.0 CoO 2 to 6.67 nm ps −1 for Li 0.6 CoO 2 ( Fig. 3b ). It is interesting that the longitudinal elastic modulus is a linear function of Li content but thermal conductivity plateaus below x =0.8 ( Fig. 3a ). The different composition dependence of the elastic constants and thermal conductivity suggests that changes in thermal conductivity with lithiation are not due to a softening of the lattice with decreasing lithium content, but rather are related to the Li x CoO 2 phase behaviour. To summarize, we experimentally show that the thermal conductivity of Li x CoO 2 , an important material for electrochemical energy storage, can be reversibly electrochemically modulated over a considerable range. Both the thermal conductivity and elastic modulus change significantly over the range of Li 1.0 CoO 2 to Li 0.6 CoO 2 , in a system which has only a 1.3% change in the unit cell volume. The mechanism of the electrochemically driven thermal conductivity change is not yet clear but may be related to the lithiation-dependent phase behaviour. TDTR measurements TDTR is used to measure the thermal conductivity of the Li x CoO 2 thin film as a function of lithiation. The TDTR measurements use an 80-MHz mode-locked Ti:sapphire laser, and the pump beam is modulated at 9.8 MHz with an electro-optical modulator. The reflectance of the probe beam is detected at the pump’s modulation frequency using a lock-in amplifier. The ratio of the in-phase to out-of-phase signal ( V in /V out ) is then fit to a thermal diffusion model. Two thermal models were used to analyse the data for the changes in reflectivity as a function of delay time: uni-directional heat flow was used to analyse the heat transfer in case of ex situ TDTR measurement, and bi-directional heat flow was used to analyse the heat transfer in case of in situ TDTR measurement setup. To rapidly measure the thermal conductivity of LiCoO 2 during lithiation and delithiation process, the V in /V out signal at 30 ps was monitored using a fixed delay stage. As shown in Fig. 2c , the voltage ratios at 30 ps were measured every 6 s and a TDTR scan over the delay range of 0–3.6 ns was conducted only every 20 min. The voltage ratio at 30 ps was converted to thermal conductivity value according to the relationship between voltage ratio and thermal conductivity. Using bi-directional thermal model, the relation between the voltage ratio and thermal conductivity can be fitted using a polynomial equation ( Supplementary Fig. 15 ). To evaluate the thermal conductivity of the Li x CoO 2 by TDTR, the thickness, thermal conductivity and heat capacity for all other layers must be known accurately. The heat capacities for Al, SiO 2 and sapphire were obtained from literature values. The thickness of the Al layer was measured using X-ray reflectometry (XRR). The thermal conductivity of Al was obtained by measuring the in-plane electrical conductivity and then the thermal conductivity was calculated from the Wiedemann–Franz law. The thickness of the SiO 2 layer deposited by PECVD was measured by XRR and its thermal conductivity was determined from TDTR measurement of a Si/SiO 2 /Al sample to be 2.8 W m −1 K −1 , a factor of 2 greater than expected. The reason for the high effective thermal conductivity of the SiO 2 layer is still under investigation. The volumetric heat capacities used are C p =3.62 J cm −3 K for Li 1.00 CoO 2 (refs 33 , 34 ) and C p =3.26 J cm −3 K for Li 0.60 CoO 2 . The volumetric heat capacity change of Li x CoO 2 with delithiation is assumed to change linearly with the number density of atoms [35] . The modelling parameters are summarized in Supplementary Tables 1 and 2 . Sample preparation The in situ TDTR liquid cell was fabricated as follows. c-Plane-oriented sapphire was used as a transparent substrate. One side of the sapphire substrate was coated with ~100 nm of SiO 2 using PECVD. Then, an ~80 nm Al layer was deposited by direct current (DC) magnetron sputtering. This Al film served as the current collector for electrochemical measurement and the optical transducer layer for TDTR measurements. Reactive RF sputtering from stoichiometric Li 1.0 Co 1.0 O 2 targets (99.7%, Kurt J. Lesker Company Ltd) was used to deposit ~500 nm of LiCoO 2 on the Al. The sputtering conditions were: room temperature substrate, argon-oxygen working pressure of 5 mTorr in a 9:1 ratio, RF power of 50 W and a target-to-substrate distance of 10 cm. At these conditions, the growth rate of LiCoO 2 is ~8 Å min −1 . Post annealing was performed to crystallize the sputtered LiCoO 2 thin film. Samples were annealed with a ramping rate of 10 °C min −1 to 500 °C in air for 1 h. The use of Al (as the current collector) limits the upper annealing temperature below its melting point of 660.4 °C. Even at temperatures below the melting point, one must be aware of possible oxidation of the Al film and interdiffusion of soluble species in the individual stack layers. Experimentally, the maximum annealing temperature on Al was limited to 500 °C. As shown in Supplementary Fig. 1 , the best electrochemical performance from LiCoO 2 was obtained with 700 °C annealing. However, the capacity of the LiCoO 2 thin film using an Al current collector starts to decrease and the resistance of the Al layer increases because of oxidation at annealing temperature greater than 500 °C ( Supplementary Fig. 2 ). After annealing, the liquid cell was assembled in a glove box (MBraun, H 2 O and O 2 <3 p.p.m.) using a Li foil (Aldrich, 99%) counter electrode and a liquid electrolyte of 1:1 ethylene carbonate (Aldrich, anhydrous, 99%) and dimethyl carbonate (Aldrich, anhydrous, 99%) containing 1 M LiClO 4 (Aldrich, battery grade, dry, 99.99%). The ex situ sample was fabricated on a Pt-coated Si wafer. The annealing temperature was 700 °C. After electrochemical lithiation and/or delithiation, an Al layer was deposited on the LiCoO 2 thin film. The Al served as the transducer for TDTR measurement. Samples were characterized in air. Electrochemical characterization Supplementary Fig. 3 shows cycling data of the 500 °C annealed LiCoO 2 thin film. The LiCoO 2 was pre-cycled three times to establish a stable intercalation reaction before TDTR measurements. Supplementary Fig. 3A shows the cyclic voltammetry (CV) data over ten cycles. In the first scan, well-defined anodic and cathodic peaks are seen around 3.93 and 3.88 V, respectively. The redox couple around 3.9 V is attributed to a first-order phase transition between the H1 and H2 hexagonal phases (two-phase co-existence region). There is a minor anodic peak around 3.75 V as well which indicates that LiCoO 2 annealed at 500 °C has a mixture of well-ordered HT-LiCoO 2 (LiCoO 2 prepared at high temperature) and LT-LiCoO 2 (LiCoO 2 prepared at low temperature) (ref. 36 ). Figure 1b shows the randomly oriented polycrystalline structure of the LiCoO 2 . Even though the LiCoO 2 is not fully crystallized into the HT phase at 500 °C, clear redox couples for Li intercalation in the CV scan and a potential plateau around 3.9 V are observed during TDTR measurements. Supplementary Fig. 4 shows the cycling data and CV curve of the 700 °C annealed LiCoO 2 thin film. Well-defined anodic and cathodic peaks at 3.93 and 3.88 V are observed, and the capacity fade is reduced from the 500 °C annealed film. Lithiation determination In Fig. 3 , the irreversible capacity loss is accounted for by assuming that the as-sputtered film is Li 1.0 CoO 2 . During delithiation to 4.2 V, the total charge transfer is measured, and assuming no capacity loss upon delithiation, the charge transfer corresponds to a composition of Li 0.6 CoO 2 . Then, we assume lithiation to 3.0 V results in formation of Li 1.0 CoO 2 (ref. 37 ). Because of irreversible capacity loss, if the total charge transfer is measured during lithiation, the film composition would be Li 0.9 CoO 2 , which is not reasonable at 3.0 V versus Li. The irreversible capacity loss is corrected for by stretching the lithiation data uniformly over the range of Li 0.6 CoO 2 to Li 1.0 CoO 2 . This approach assumes all the irreversible capacity loss occurs during the lithiation cycle. Although this is not rigorously true, assuming the capacity loss occurs uniformly or entirely during the delithiation cycle requires a more complex correction function, which is no more likely to be valid, so the simplest data correction possible was applied. Crystal structure analysis For cross-sectional TEM studies, the LiCoO 2 film was deposited on top of 30 nm of Al which was deposited on top of 500 nm of SiO 2 . A 100-oriented silicon substrate was used, and the sample was annealed at 500 °C following the same procedure as for the TDTR samples. The thin film was cut normal to the 110 plane of silicon substrate into a thin slice. This was followed by mechanical polishing to a thickness of approximately 20 μm. The sample was thinned to electron transparency by ion milling using 3.5 and 2.0 kV Ar ions at a glancing angle of ±8°. High-resolution TEM (HRTEM) images and diffraction patterns were recorded using a JEOL 2100 TEM equipped with a LaB 6 gun and operated at 200 kV. In the low-magnification TEM image presented in Supplementary Fig. 5A, it can be seen that the film has a columnar structure with a relatively uniform thickness of 260 nm. Supplementary Fig. 5B–D shows a HRTEM image of the 500 °C annealed LiCoO 2 . Lattice fringes are resolved. They appear randomly oriented, consistent with the electron diffraction data. Crystalline grains as large as 10 nm can be identified in the HRTEM images. The grains appear elongated along the growth direction. To verify further the structure of LiCoO 2 , electron diffraction analysis was performed using an electron beam 140 nm in diameter formed in nano-beam diffraction mode. Diffraction patterns were recorded by placing the beam directly on the LiCoO 2 film. Figure 1b inset shows an example of diffraction pattern recorded from the LiCoO 2 film. To index the diffraction ring patterns, the intensities of the recorded diffraction pattern are radially averaged around the centre of the diffraction patterns. The averaged intensity profile in Supplementary Fig. 6 was then used to identify the structure of LiCoO 2 . The major peaks correspond to the rhombohedral structure of LiCoO 2 . The diffraction peaks indicated by red arrows are not consistent with the rhombohedral structure. These diffraction peaks can originate from other phases formed in the LiCoO 2 film during annealing process. Intensity peaks marked by orange arrows are artefacts resulting from partially blocked central beam by the beam stop. Supplementary Fig. 7 shows a HRTEM image of the LiCoO 2 film annealed at 700 °C in air. The grain size is larger than for the 500 °C annealed LiCoO 2 film. Supplementary Fig. 8 presents X-ray diffraction from LiCoO 2 deposited on a Si/SiO 2 /Al substrate after annealing at 500 °C. The JCPDS data for LiCoO 2 are shown as vertical lines. The diffraction indicates the structure is (101) and (104) textured, as the (003) diffraction, which for a powder sample is slightly stronger than the (104) peak, is nearly missing. How to cite this article: Cho, J. et al . Electrochemically tunable thermal conductivity of lithium cobalt oxide. Nat. Commun. 5:4035 doi: 10.1038/ncomms5035 (2014).